Integrin-linked kinase mediates force transduction in cardiomyocytes by modulating SERCA2a/PLN function Human dilated cardiomyopathy (DCM) manifests as a profound reduction in biventricular cardiac function that typically progresses to death or cardiac transplantation. There is no effective mechanism-based therapy currently available for DCM, in part because the transduction of mechanical load into dynamic changes in cardiac contractility (termed mechanotransduction) remains an incompletely understood process during both normal cardiac function and in disease states. Here we show that the mechanoreceptor protein integrin-linked kinase (ILK) mediates cardiomyocyte force transduction through regulation of the key calcium regulatory protein sarcoplasmic/endoplasmic reticulum Ca 2+ ATPase isoform 2a (SERCA-2a) and phosphorylation of phospholamban (PLN) in the human heart. A non-oncogenic ILK mutation with a synthetic point mutation in the pleckstrin homology-like domain (ILK R211A ) is shown to enhance global cardiac function through SERCA-2a/PLN. Thus, ILK serves to link mechanoreception to the dynamic modulation of cardiac contractility through a previously undiscovered interaction with the functional SERCA-2a/PLN module that can be exploited to rescue impaired mechanotransduction in DCM. Dilated cardiomyopathy (DCM) is defined by the presence of left ventricular (LV) dilatation and systolic dysfunction [1] . Next-generation sequencing has revealed considerable genotypic heterogeneity among the common cardiomyopathic phenotypes (hypertrophic, dilated, restrictive and arrhythmogenic RV dysplasia), although mutations in cytoskeletal, Z-disk, mitochondrial and calcium handling proteins are prominently featured in the dilated phenotype [1] , [2] . The profound loss of cardiac function present in advanced DCM points to disruption in the molecular pathways that link the reception of mechanical stress to coherent changes in cardiac contractility. Advances in the molecular therapy of DCM are likely to converge on cardiomyocyte calcium regulation, given its critical role in contractility and its dysregulation in diverse cardiac diseases [3] . The key calcium regulatory protein in heart is sarcoplasmic/endoplasmic reticulum Ca 2+ ATPase isoform 2a (SERCA-2a). Phospholamban (PLN) is the principal physiological inhibitor of SERCA-2a, and phosphorylation of PLN (pPLN) at residues Serine 16 or Threonine 17 enhances SERCA-2a function by decreasing the efficacy of PLN-mediated inhibition [4] . The major phosphatase-dephosphorylating PLN is protein phosphatase 1 (PP1) and the activity of this enzyme is increased in failing human hearts [5] , [6] . Excessive PP1 activation is opposed by its endogenous inhibitor, PP1 inhibitor-1, so that normalization of PP1 activity through upregulation of PP1 inhibitor-1 represents a novel molecular therapy directed to improve calcium regulation in heart failure [5] . Importantly, various calcium cycling proteins that modulate SERCA-2a/PLN function are now addressable by gene therapy [5] , [7] , [8] . Nevertheless, the upstream molecular signals linked to impaired SERCA-2a/PLN function in heart failure are unknown. The contractile sarcomeric units within the cardiomyocyte are delimited by the Z-disks that contain a large network of interacting proteins that ensure force transduction from the sarcomeric units to the sarcolemma, the extracellular matrix and to adjacent cardiomyocytes [9] . Integrin-linked kinase (ILK) is highly expressed in the sarcomeric Z-disk costamere (region of close intermyocyte linkage) and is a critical component of the protein scaffold required for integrated force transduction during normal cardiac function [10] , [11] , [12] . Indeed, ILK mutations have been reported in human DCM [1] , [13] and conditional gene deletion of Ilk leads to neonatal cardiomyopathy in mouse [14] . Conversely, tetralogy of Fallot (TF) represents a compensatory type of right ventricular (RV) hypertrophy featuring preserved RV function and structure in association with elevated levels of ILK expression [15] . Here we show that ILK mediates cardiomyocyte force transduction through regulation of the key calcium regulatory protein SERCA-2a and the phosphorylation of PLN in the human heart. The ILK–SERCA2a–PLN interaction provides an elegant mechanism for transduction of mechano- and stress reception into dynamic, calcium-mediated changes in cardiomyocyte contractility, revealing ILK as a novel, therapeutically addressable target applicable to a wide range of heart diseases. ILK colocalizes with SERCA-2a and PLN at the Z-disk SERCA-2a is located in the sarcoplasmic reticulum (SR) that comprises the main calcium release units that are concentrated at Z lines [16] . Confocal microscopy in human myocardial samples from patients with TF revealed Z-disk colocalization of endogenous ILK with SERCA-2a and PLN and the Z-disk protein α-actinin, whereas there was no spatial overlap detectable of ILK or SERCA-2a with the sacromeric protein Troponin T ( Fig. 1a ). In contrast, myocardium from patients with advanced DCM exhibited conspicuous loss of colocalization of ILK with SERCA-2a and with α-actinin, as well as disruption of the normal striated pattern of sarcomeric Troponin T staining ( Fig. 1b ). Loss of Z-disk architecture was also evident in the DCM myocardium, a finding that is recapitulated in isolated cardiomyocytes derived from induced pluripotent stem cells in patients with DCM [17] . The interaction of ILK and SERCA-2a was further probed in ILK immunoprecipitates (IPs) from the hearts of mice with transgenic myocardial overexpression of wild-type ILK (ILK WT ) [15] , which revealed co-immunoprecipitation (co-IP) of ILK with SERCA-2a confirmed using mass spectrometry ( Supplementary Fig. 1a,b ). Reciprocal co-IP analyses confirmed the binding of ILK with PLN, the principal physiological inhibitor of SERCA-2a, and binding of PLN with SERCA-2a ( Supplementary Fig. 1c ). Thus, the interaction of ILK with the SERCA-2a–PLN protein complex within Z-disks and costameric structures provides a potential target for disruption under disease conditions in which intermyocytic adhesive interactions are compromised [18] . 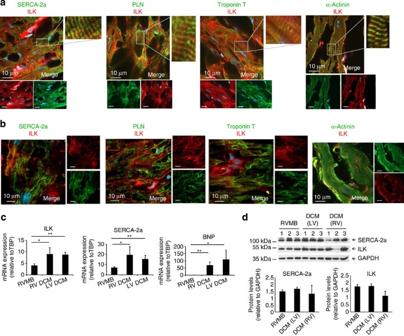Figure 1: ILK and SERCA-2a colocalize in human myocardium. (a) Representative confocal micrographs of cryosectioned RV sample from a patient with TF.Left panel, immunostaining for ILK (red) merged with SERCA-2a (green);left middle panel, ILK (red) merged with PLN (green);right middle panel,ILK (red) merged with Troponin T (green); right panel, ILK (red) merged with α-actinin. ILK, SERCA-2a PLN and α-actinin colocalize in Z-disks, whereas Troponin T shows sarcomeric localization. Nuclei were detected with 4,6-diamino-2-phenylindole staining (blue). Scale bar, 10 μm. The windows show the corresponding boxed areas at × 3 magnification. Confocal micrographs are representative of three different patients with TF. (b) Representative confocal micrographs of cryosectioned RV from a patient with advanced DCM demonstrating disruption of the normal striated pattern of sarcomeric Troponin T staining, localization of ILK staining to cell surface and loss of colocalization of ILK with SERCA-2a, PLN and α-actinin at the Z-disks. Confocal micrographs are representative of five different patients with DCM. (c) Real-time quantitative PCR of ILK, SERCA-2a and BNP levels in RV and LV myocardium from patients with RVMB and DCM. Expression levels are presented as the ratio over TATA-binding protein (TBP). Bars represent the mean±s.e.m. of values obtained from six RVMB and nine DCM samples. *P<0.05, **P<0.01, by Student’st-test. (d)Upper panel, western blot analysis of heart lysates acquired during repair of RVMB (n=3 patients) and from excised RV and LV myocardium during cardiac transplantation for DCM (n=3 patients). The blot was probed for SERCA-2a and ILK. GAPDH was used as a loading control.Lower panel, corresponding protein expression levels of SERCA-2a and ILK determined by densitometry of western blots and normalized to GAPDH.P=NS for all comparisons. Figure 1: ILK and SERCA-2a colocalize in human myocardium. ( a ) Representative confocal micrographs of cryosectioned RV sample from a patient with TF. Left panel , immunostaining for ILK (red) merged with SERCA-2a (green); left middle panel , ILK (red) merged with PLN (green); right middle panel, ILK (red) merged with Troponin T (green); right panel, ILK (red) merged with α-actinin. ILK, SERCA-2a PLN and α-actinin colocalize in Z-disks, whereas Troponin T shows sarcomeric localization. Nuclei were detected with 4,6-diamino-2-phenylindole staining (blue). Scale bar, 10 μm. The windows show the corresponding boxed areas at × 3 magnification. Confocal micrographs are representative of three different patients with TF. ( b ) Representative confocal micrographs of cryosectioned RV from a patient with advanced DCM demonstrating disruption of the normal striated pattern of sarcomeric Troponin T staining, localization of ILK staining to cell surface and loss of colocalization of ILK with SERCA-2a, PLN and α-actinin at the Z-disks. Confocal micrographs are representative of five different patients with DCM. ( c ) Real-time quantitative PCR of ILK, SERCA-2a and BNP levels in RV and LV myocardium from patients with RVMB and DCM. Expression levels are presented as the ratio over TATA-binding protein (TBP). Bars represent the mean±s.e.m. of values obtained from six RVMB and nine DCM samples. * P <0.05, ** P <0.01, by Student’s t- test. ( d ) Upper panel , western blot analysis of heart lysates acquired during repair of RVMB ( n =3 patients) and from excised RV and LV myocardium during cardiac transplantation for DCM ( n =3 patients). The blot was probed for SERCA-2a and ILK. GAPDH was used as a loading control. Lower panel , corresponding protein expression levels of SERCA-2a and ILK determined by densitometry of western blots and normalized to GAPDH. P= NS for all comparisons. Full size image On the basis of the finding of ILK–SERCA-2a–PLN interaction, the possibility was examined that ILK may control the expression levels of ATP2A , which encodes SERCA-2a, in human myocardium in various cardiac diseases with preserved or compromised ventricular function. The gene expression levels of Ilk determined using quantitative real time–PCR (qRT–PCR) were significantly increased in the RV and LV samples from DCM patients compared with those from patients with ventricular septal defect with RV muscle bundles (RVMB) that represent normal RV/LV function ( Fig. 1c ). Expression of ATP2A (SERCA-2a) was similarly upregulated. As expected, B-type natriuretic peptide precursor ( NPPB ), a biomarker of heart failure, was significantly increased ( Fig. 1c ). The signal responsible for increased ILK and SERCA-2a mRNA expression in DCM is unknown but may result from increased mechanical stretch secondary to ventricular dilatation and transduction through integrin-dependent signalling, analogous to upregulated ILK transcription following integrin engagement described in ovarian cancer cells [19] . In contrast, the corresponding protein expression levels of ILK and SERCA-2a were unchanged in DCM samples ( Fig. 1d ), suggesting that ILK and SERCA-2a protein expression levels are regulated postranscriptionally in DCM. Similarly, SERCA-2a protein levels have been reported as unchanged or decreased in heart failure [20] but are typically observed to be unchanged in DCM [21] , [22] . ILK activates SERCA-2a/PLN through CaMKII Since ILK and SERCA-2a form a putative functional module, we asked whether ILK upregulation affects SERCA-2a/PLN function in human cardiomyocytes derived from induced pluripotent stem cells (iPSC-CMs). Unlike most experimental cardiomyocyte preparations, iPSC-CMs maintain a robustly contractile phenotype in vitro [23] , [24] . Transduction of ILK WT caused an increase in SERCA-2a levels and in phosphorylation of PLN on Thr17 (pPLN; Fig. 2a ). Inactivation of GSK-3β through phosphorylation at Ser9 (pGSK-3β) is cytoprotective in the myocardium [25] , [26] and is a common readout of ILK activation [27] , [28] . ILK overexpression caused an increase in phosphorylation of GSK-3β, whereas ILK knockdown by short interfering RNA (siRNA) caused a relative de-phosphorylation of GSK-3β ( Fig. 2a,b ). Thus, ILK overexpression results in a signalling profile consistent with activation of the PLN/SERCA-2a regulatome [5] . Since ILK is a potential oncogene, we tested in parallel the ILK mutant with a synthetic arginine (R) to alanine (A) point mutation in the PH domain (ILK R211A ) [29] . This mutant is deficient in membrane binding and is non-oncogenic [15] , [29] and is therefore a potential gene therapy candidate. The effects of ILK R211A transduction in iPSC-CMs were the same as those of ILK WT , featuring increased levels of SERCA-2a, pPLN and pGSK-3β ( Fig. 2a ). Since pPLN (Thr17) is a unique target of calcium/calmodulin-dependent protein kinase II (CaMKII) [30] , [31] , we tested for and confirmed the induction of the principal activating phosphorylation site of CaMKII at 286 (pCaMKII) upon transduction of ILK WT and ILK R211A ( Fig. 2a ). Conversely, transduction of ILK-targeted siRNA resulted in decreased phosphorylation of CaMKII and PLN and a reduction in SERCA-2a protein levels, thus positioning CaMKII as a downstream target of endogenous ILK ( Fig. 2b ). Further, the CaMKII inhibitor KN-93 but not the inactive analogue KN-92 reduced the levels of pCaMKII, SERCA-2a and pPLN in a concentration-dependent manner ( Fig. 2c ). 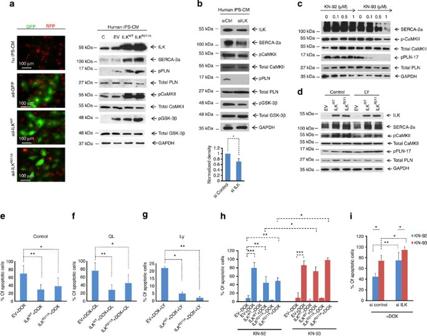Figure 2: Both ILKWTand ILKR211Aupregulate the protein expression of SERCA-2a and phospho-PLN17 in human iPSC-derived cardiomyocytes. Left panel, fluorescence microscopy images of human iPSC-CMs transduced with adenoviral green-fluorescent protein (GFP)-linked vector (ad-GFP or EV-empty vector), ad-ILKWTand the mutant ILK (ad-ILKR211A). Green fluorescence indicates efficient transduction of ILK constructs. The cells also express red-fluorescent protein (RFP) and blasticidin resistance gene under the control of the alpha-myosin heavy chain promoter enabling purification and identification. Scale bar, 100 μm.Right panel, western blot analysis of ILK, SERCA-2a and phosphorylated and total forms of PLN, CaMKII and GSK-3β in human iPSC-CMs transduced with ad-ILKWT(ILKWT), ad-ILKR211A(ILKR211A), empty vector (EV) or control, non-transduced cells (c). GAPDH was used as a loading control. Western blot is representative of more than five experiments. (b)Upper panel, lysates of human iPSC-CMs transduced with ILK-targeted siRNA (siILK) compared with that using control, scrambled siRNA (siCtrl).Lower panel, quantitative analysis of normalized ILK protein expression levels in human iPSC-CMs transduced with siILK versus siControl. Values shown represent five independent experiments. Error bars represent mean±s.e.m. (c) Representative immunoblot for cell lysates of human iPSC-CMs treated for 24 h with various indicated concentrations of specific CaMKII inhibitor KN-93 and the inactive analogue KN-92. (d) Western blot analysis of indicated targets in human iPSC-CMs following treatment with 30 μM of PI3K inhibitor LY294002 (LY) for 24 h. (e) Percentage of TUNEL-labelled human iPSC-CMs after adenoviral infection treated for 24 h with 1 μM of DOX. *P<0.05, **P<0.01, by Student’st-test. Percentage of TUNEL-labelled human iPSC-CMs after adenoviral infection and following treatment with 20 μM of ILK kinase inhibitor QLT0267 (f) added 1 h prior exposure to 1 μM of DOX. *P<0.05, **P<0.01, by Student'st-test, (g) and following treatment with 30 μM of PI3K inhibitor LY294002 (LY). *P<0.05, **P<0.01, by Student'st-test. (h) Percentage of TUNEL-labelled human iPSC-CMs treated for 24 h with 1 μM of KN-93 or KN-92 as a control, added 1 h before treatment with 1 μM of DOX (+DOX) versus untreated cells (−DOX). *P<0.05, **P<0.01, ***P<0.001, by Student’st-test. (i) Percentage of TUNEL-labelled human iPSC-CMs transduced with siILK compared with that using control, scrambled siRNA (siCtrl) following treatment with 1 μM of KN-93 or KN-92. *P<0.05, **P<0.01, ***P<0.001 by Student’st-test. Figure 2: Both ILK WT and ILK R211A upregulate the protein expression of SERCA-2a and phospho-PLN17 in human iPSC-derived cardiomyocytes. Left panel , fluorescence microscopy images of human iPSC-CMs transduced with adenoviral green-fluorescent protein (GFP)-linked vector (ad-GFP or EV-empty vector), ad-ILK WT and the mutant ILK (ad-ILK R211A ). Green fluorescence indicates efficient transduction of ILK constructs. The cells also express red-fluorescent protein (RFP) and blasticidin resistance gene under the control of the alpha-myosin heavy chain promoter enabling purification and identification. Scale bar, 100 μm. Right panel , western blot analysis of ILK, SERCA-2a and phosphorylated and total forms of PLN, CaMKII and GSK-3β in human iPSC-CMs transduced with ad-ILK WT (ILK WT ), ad-ILK R211A (ILK R211A ), empty vector (EV) or control, non-transduced cells ( c ). GAPDH was used as a loading control. Western blot is representative of more than five experiments. ( b ) Upper panel , lysates of human iPSC-CMs transduced with ILK-targeted siRNA (siILK) compared with that using control, scrambled siRNA (siCtrl). Lower panel , quantitative analysis of normalized ILK protein expression levels in human iPSC-CMs transduced with siILK versus siControl. Values shown represent five independent experiments. Error bars represent mean±s.e.m. ( c ) Representative immunoblot for cell lysates of human iPSC-CMs treated for 24 h with various indicated concentrations of specific CaMKII inhibitor KN-93 and the inactive analogue KN-92. ( d ) Western blot analysis of indicated targets in human iPSC-CMs following treatment with 30 μM of PI3K inhibitor LY294002 (LY) for 24 h. ( e ) Percentage of TUNEL-labelled human iPSC-CMs after adenoviral infection treated for 24 h with 1 μM of DOX. * P <0.05, ** P <0.01, by Student’s t- test. Percentage of TUNEL-labelled human iPSC-CMs after adenoviral infection and following treatment with 20 μM of ILK kinase inhibitor QLT0267 ( f ) added 1 h prior exposure to 1 μM of DOX. * P <0.05, ** P <0.01, by Student's t- test, ( g ) and following treatment with 30 μM of PI3K inhibitor LY294002 (LY). * P <0.05, ** P <0.01, by Student's t- test. ( h ) Percentage of TUNEL-labelled human iPSC-CMs treated for 24 h with 1 μM of KN-93 or KN-92 as a control, added 1 h before treatment with 1 μM of DOX (+DOX) versus untreated cells (−DOX). * P <0.05, ** P <0.01, *** P <0.001, by Student’s t- test. ( i ) Percentage of TUNEL-labelled human iPSC-CMs transduced with siILK compared with that using control, scrambled siRNA (siCtrl) following treatment with 1 μM of KN-93 or KN-92. * P <0.05, ** P <0.01, *** P <0.001 by Student’s t- test. Full size image The increase in SERCA-2a protein levels following transduction of ILK WT and ILK R211A in iPSC-CMs results from post-transcriptional regulation since SERCA-2a transcript levels, as determined using qPCR, were unchanged ( Supplementary Fig. 2 ). One possibility is that SERCA-2a is stabilized or protected from degradation by binding to ILK, the expression of which is concomitantly elevated following ILK WT and ILK R211A transductions. Consistent with this possibility, the capacity of ILK R211A to co-IP with SERCA-2a was determined in heart lysates from mice with transgenic myocardial overexpression of ILK R211A ( Supplementary Figs 1 and 3 ). Thus, both ILK variants (ILK WT and ILK R211A ) exhibit co-IP with SERCA-2a and reciprocal co-IP with PLN. Samples from littermate controls conveying endogenous expression levels also revealed clearly discernible co-IP between ILK, SERCA-2a and PLN ( Supplementary Fig. 3a,b ). Further, the ILK–SERCA-2a interaction was demonstrated after equalization of the amounts of immunoprecipitated ILK before immunoblotting with anti-SERCA-2a antibodies ( Supplementary Fig. 3c ), indicating that these interactions were not simply the result of high transgenic levels of ILK expression. Our results suggest that the ILK R211A mutation retains the molecular scaffolding properties of ILK WT sufficient for binding to the PLN/SERCA-2a regulatome, and that overexpression of ILK WT or ILK R211A results in increased levels of SERCA-2a through a binding-dependent mechanism. ILK activates SERCA-2a/PLN via scaffolding mechanism There is debate as to whether ILK functions as a serine–threonine kinase [28] , or alternatively, as a scaffolding protein [32] , to mediate adhesion-dependent integrin signalling. Activation of ILK kinase function occurs downstream of phosphatidylinositide 3-kinase (PI3K) activation through binding of the phosphoinositide phospholipid product of PI3K, PI 3,4,5-triphosphate, to the pleckstrin-homology domain of ILK [28] , [33] . Many cancers harbour oncogenic mutations or amplifications in components of the PI3K pathway that are subject to hyperactivation [34] . The expression levels of SERCA-2a and the phosphorylation profile of PLN (decreasing the efficacy of PLN-mediated inhibition of SERCA-2a function) resulting from ILK WT and ILK R211A overexpression were not attenuated by the PI3K inhibitor LY294002 ( Fig. 2d ). Thus, in the human cardiomyocyte, the effects of ILK overexpression on PLN/SERCA-2a function do not depend upon canonical PI3K-mediated activation. Rather, enhancement of PLN/SERCA-2a function by ILK WT/R211A appears to be dependent upon the previously documented adaptor functions of ILK [32] , [35] . ILK WT/R211A mitigates DOX cardiotoxicity Doxorubicin (DOX) is an effective and frequently used chemotherapeutic agent for various malignancies, which causes both an acute and late-onset, dose-limiting cardiomyopathy [36] , [37] , [38] , in part, as a result of cumulative apoptotic myocyte loss [39] , [40] . Transduction of ILK WT and ILK R211A caused a significant reduction in DOX-induced apoptosis ( Fig. 2e ). The requirement for inherent ILK kinase catalytic activity to mediate cytoprotection against DOX cardiotoxicity was further tested using the ILK kinase inhibitor QLT0267 (ref. 28 ; Fig. 2f ) and the PI3K inhibitor LY294002 ( Fig. 2g ). The anti-apoptotic effects of ILK (WT and R211A) were not abrogated by the PI3K inhibitor LY294002 or by ILK kinase inhibition, suggesting that the ILK-mediated prosurvival effect depends upon a scaffolding mechanism and not upon PI3K or ILK kinase activation. In fact, there is an apparent protective effect of LY294002 in both the presence and absence of ILK transductions suggesting that PI3K activation, through an alternative mechanism, is detrimental to DOX-induced apoptosis resistance. In contrast, the CaMKII inhibitor KN-93, but not the inactive analogue KN-92, abrogated ILK-mediated apoptosis protection against DOX, revealing the requirement for CaMKII activation ( Fig. 2h ). Silencing of endogenous ILK potentiated the extent of DOX-induced apoptosis in the presence of both CaMKII inhibitor KN-93 and the inactive analogue KN-92 ( Fig. 2i ). However, the extent of apoptosis reduction was significantly less in the presence of the CaMKII inhibitor KN-93, positioning CaMKII downstream of ILK in a prosurvival pathway ( Fig. 2i ). These results point to a novel cytoprotective pathway in the cardiomyocyte activated by ILK overexpression and requiring pCaMKII, and are consistent with the documented cytoprotective effects of CaMKII activation and Thr17 phosphorylation of PLN against myocyte ischemic injury [20] . ILK modulates calcium transient profiles through SERCA-2a Increased ILK-mediated expression of SERCA-2a and pPLN is predictive of enhanced SR Ca 2+ reuptake and diastolic relaxation. Accordingly, cardiomyocyte calcium transients were measured in rhodamine-3-loaded human iPSC-CMs using laser confocal microscopy. The spontaneous firing rate of ventricular myocytes is directly related to the rate of Ca 2+ reuptake by SR as measured by the monoexponential Ca 2+ decay constant tau ( τ ) and is mainly dependent upon the function of SERCA-2a [41] . ILK (both WT and R211A)-transduced iPSC-CMs showed a significantly reduced τ ( Fig. 3a,b ) and an increased spontaneous beat rate compared with vector-only control cells ( Fig. 3c ), corresponding to an increase in SERCA-2a function. CaMKII activation increases SERCA-2a function leading to increased SR Ca 2+ content [42] . Accordingly, the effects of ILK overexpression on SR Ca 2+ content were determined using caffeine to effect SR Ca 2+ release through ryanodine receptor Ca 2+ channels [43] ( Supplementary Fig. 4 ). Indeed, SR Ca 2+ content increased following transduction of ILK WT and ILK R211A , in line with the ILK-regulated activation of CaMKII- and ILK-dependent increase in SERCA-2a/PLN function [44] . 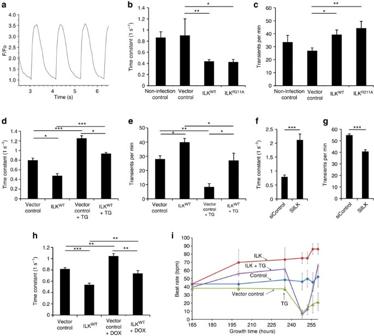Figure 3: Modulation of spontaneous beat rate and Ca2+reuptake kinetics in human iPSC-CMs by ILK is SERCA-2a-dependent. (a) Representative tracing of calcium transients measured using line scan confocal microscopy in Rhod-3-loaded iPSC-CMs. (b) Transduction of ILKWT(individual cardiomyocytes,(n=7)) and ILKR211A(n=3) in iPSC-CMs for 24 h decreased the time constantτcompared with vector control (n=9). *P<0.05, **P<0.01, by Student’st-test. (c) Transduction of ILKWT(n=7) and ILKR211A(n=5) in iPSC-CMs for 24 h increased the number of spontaneous calcium transients per minute compared with vector control (n=7). *P<0.05, **P<0.01, by Student’st-test. (d) Addition of SERCA-specific inhibitor TG (1 μM) to ILKWT(n=4) and vector control (n=3) transduced iPSC-CMs increased the time constantτcompared with controls (Vector Controln=5; ILKWTn=5). *P<0.05, ***P<0.001, by Student’st-test. (e) Treatment with TG in ILKWTtransduced (n=4) and vector control (n=3) iPSC-CMs decreased the number of spontaneous calcium transients per minute compared with controls (Vector Controln=5; ILKWTn=5). *P<0.05, **P<0.01, by Student’st-test. (f) Treatment with siILK (n=9) in iPSC-CMs for 48 h increased the time constantτcompared with scrambled siRNA control (n=6). ***P<0.001, by Student’st-test. (g) Treatment with siILK (n=9) in iPSC-CMs for 48 h decreased the number of spontaneous calcium transients per minute compared with scrambled siRNA control (n=8). ***P<0.001, by Student’st-test. (h) Treatment with DOX at 1 μM for 24 h in ILKWTtransduced (n=4) and vector control (n=4) iPSC-CMs increased the time constantτcompared with controls (Vector Controln=3; ILKWTn=5). **P<0.01, ***P<0.001, by Student’st-test. (i) Transduction with ILKWT(shown at time point A) resulted in faster baseline beat rate compared with vector control (Student’st-testP<0.02) as determined by impedance measurements acquired during at least 10 days in iPSC-CMs. The addition of TG (1 μM) at time point B reduced the beat rate in all groups (Student’st-testP<0.02), which recovered to pre-treatment beat rate in ILKWTtransduced iPSC-CMs (Student’st-testP<0.02) compared with vector control (minimum of three impedance measurements per time point). Error bars represent mean±s.e.m. Figure 3: Modulation of spontaneous beat rate and Ca 2+ reuptake kinetics in human iPSC-CMs by ILK is SERCA-2a-dependent. ( a ) Representative tracing of calcium transients measured using line scan confocal microscopy in Rhod-3-loaded iPSC-CMs. ( b ) Transduction of ILK WT (individual cardiomyocytes, (n =7)) and ILK R211A ( n =3) in iPSC-CMs for 24 h decreased the time constant τ compared with vector control ( n =9). * P <0.05, ** P <0.01, by Student’s t- test. ( c ) Transduction of ILK WT ( n =7) and ILK R211A ( n =5) in iPSC-CMs for 24 h increased the number of spontaneous calcium transients per minute compared with vector control ( n =7). * P <0.05, ** P <0.01, by Student’s t- test. ( d ) Addition of SERCA-specific inhibitor TG (1 μM) to ILK WT ( n =4) and vector control ( n =3) transduced iPSC-CMs increased the time constant τ compared with controls (Vector Control n =5; ILK WT n =5). * P <0.05, *** P <0.001, by Student’s t- test. ( e ) Treatment with TG in ILK WT transduced ( n =4) and vector control ( n =3) iPSC-CMs decreased the number of spontaneous calcium transients per minute compared with controls (Vector Control n =5; ILK WT n =5). * P <0.05, ** P <0.01, by Student’s t- test. ( f ) Treatment with siILK ( n =9) in iPSC-CMs for 48 h increased the time constant τ compared with scrambled siRNA control ( n =6). *** P <0.001, by Student’s t- test. ( g ) Treatment with siILK ( n =9) in iPSC-CMs for 48 h decreased the number of spontaneous calcium transients per minute compared with scrambled siRNA control ( n =8). *** P <0.001, by Student’s t- test. ( h ) Treatment with DOX at 1 μM for 24 h in ILK WT transduced ( n =4) and vector control ( n =4) iPSC-CMs increased the time constant τ compared with controls (Vector Control n =3; ILK WT n =5). ** P <0.01, *** P <0.001, by Student’s t- test. ( i ) Transduction with ILK WT (shown at time point A) resulted in faster baseline beat rate compared with vector control (Student’s t -test P <0.02) as determined by impedance measurements acquired during at least 10 days in iPSC-CMs. The addition of TG (1 μM) at time point B reduced the beat rate in all groups (Student’s t -test P <0.02), which recovered to pre-treatment beat rate in ILK WT transduced iPSC-CMs (Student’s t -test P <0.02) compared with vector control (minimum of three impedance measurements per time point). Error bars represent mean±s.e.m. Full size image The addition of the SERCA-specific inhibitors thapsigargin (TG) and cyclopiazonic acid (not shown) increased τ and reduced the cardiomyocyte firing rate ( Fig. 3d,e ), although the TG-induced changes in both τ and beat rate were reduced or nullified by ILK WT overexpression, respectively ( Fig. 3d,e ). Conversely, ILK-specific siRNA caused a decrease in the firing rate and an increase in τ ( Fig. 3f,g ). SERCA-2a is a molecular target in DOX toxicity [45] . DOX (1 μM) caused an increase in τ (that is, slower Ca 2+ reuptake), which was reversed by adenoviral transduction of ILK WT ( Fig. 3h ). Together, these results are consistent with ILK-mediated, SERCA-2a- and pPLN-dependent increased rate of SR calcium uptake. The long-term (>10 days) beat rate response to the SERCA inhibitor TG in iPSC-CMs was determined by measurements of electrical impedance using the xCELLigence RTCA Cardio System [46] , [47] . Consistent with the calcium transient profiles, transduction of ILK WT resulted in a faster baseline cardiomyocyte firing rate compared with untreated cells and to vector-only transduced controls ( Fig. 3i ). TG significantly decreased the spontaneous firing rates with incomplete recovery after 30 h in vector-only transduced control cells. However, the recovery time to pre-TG baseline was accelerated by ILK transduction, consistent with increased ILK-mediated SERCA-2a- and pPLN-dependent increased rate of SR calcium uptake. ILK R211A Tg mice exhibit increased SERCA-2a/PLN function The ILK R211A mutation has been shown to be phenotypically null in several cancer cell lines [29] , [48] , and is potentially a gene therapy candidate for heart failure indications. To test the in vivo effects of ILK R211A , we measured the protein expression profile of SERCA-2a, pPLN and pCaMKII in transgenic mice with cardiac-specific overexpression of ILK R211A (ref. 15 ; Fig. 4a ). Similar to the in vitro findings regarding ILK R211A -mediated effects in human iPSC-CMs ( Fig. 2a ), ILK R211A hearts showed activation of the SERCA-2a/pPLN regulatome relative to littermate control hearts. Alterations in pulsed-wave Tissue Doppler Indices with echocardiography (Echo) are considered as more sensitive measures of cardiac function in mouse models [49] and in patients compared with conventional M mode Echo [50] , [51] . Remarkably, ILK R211A hearts exhibited an increased baseline LV global contractility relative to that of littermate control hearts evident by a lower mean performance index (also called Tei index), a measure of global systolic and diastolic functions ( Fig. 4b ). 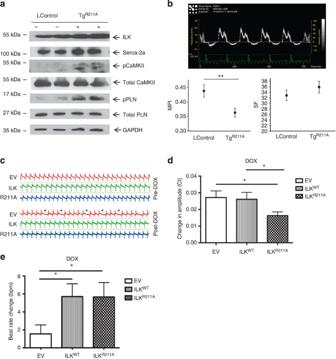Figure 4: Increased expression levels of SERCA-2a and pPLN improve both heart functionin vivoand cardiomyocyte contractilityin vitro. (a) Western blot analysis of heart lysates from 2-month-old TgR211Atransgenic mice (+) (n=2) and their littermate controls (−) (n=2) probed for ILK, SERCA-2a, pCaMKII, pPLN, total PLN and CaMKII. GAPDH was used as a loading control. (b)Upper panel, representative pulsed wave Doppler recordings taken at the mitral valve (MV). Tei index is calculated as: (isovolumic contraction time+isovolumic relaxation time)/LV ejection time (LVET). Isovolumic contraction time+isovolumic relaxation time variable is calculated as the time difference between MV closure and MV opening (MVC−MVO) minus LVET. Time intervals measured in milliseconds.Lower panels, Tei index or left ventricular mean performance index (MPI) and shortening fraction (SF) measured in ILKR211Atransgenic mice (TgR211A;n=4) and littermate controls (LControl;n=5).Lower panel,MPI in TgR211Atransgenic mice denotes increased global LV systolic and diastolic functions. **P<0.01, by Student’st-test. There was a nonsignificant trend towards higher SF in the TgR211Agenotype. (c) Real-time impedance changes in iPSC-CMs in response to DOX (1 μM) measured using RTCA cardio instrument (see Methods section for details). Treatment effects evaluated in human iPSC-CMs transduced with ad-GFP only (EV=empty vector), ad-ILKWT(ILKWT) and ad-ILKR211A(ILKR211A). Asterisks indicate high dispersion of R–R intervals, quantitated as chaos entropy coefficients: EV=−0.09; ILK=0.396; R211A=1.96.P(Mann–Whitney,for ILK and R211A versus EV) <0.05. (d) Reduction in impedance signal amplitude denoted by cell index (CI) of iPSC-CMs with the addition of DOX; treatments same as inc, *P<0.05, by Student’st-test. (e) Changes in beat rate of iPSC-CMs with DOX; treatments same as inc. *P<0.05 by Student’st-test. Error bars represent mean±s.e.m. Figure 4: Increased expression levels of SERCA-2a and pPLN improve both heart function in vivo and cardiomyocyte contractility in vitro. ( a ) Western blot analysis of heart lysates from 2-month-old Tg R211A transgenic mice (+) ( n =2) and their littermate controls (−) ( n =2) probed for ILK, SERCA-2a, pCaMKII, pPLN, total PLN and CaMKII. GAPDH was used as a loading control. ( b ) Upper panel , representative pulsed wave Doppler recordings taken at the mitral valve (MV). Tei index is calculated as: (isovolumic contraction time+isovolumic relaxation time)/LV ejection time (LVET). Isovolumic contraction time+isovolumic relaxation time variable is calculated as the time difference between MV closure and MV opening (MVC−MVO) minus LVET. Time intervals measured in milliseconds. Lower panels , Tei index or left ventricular mean performance index (MPI) and shortening fraction (SF) measured in ILK R211A transgenic mice (Tg R211A ; n =4) and littermate controls (LControl; n =5). Lower panel, MPI in Tg R211A transgenic mice denotes increased global LV systolic and diastolic functions. ** P <0.01, by Student’s t- test. There was a nonsignificant trend towards higher SF in the Tg R211A genotype. ( c ) Real-time impedance changes in iPSC-CMs in response to DOX (1 μM) measured using RTCA cardio instrument (see Methods section for details). Treatment effects evaluated in human iPSC-CMs transduced with ad-GFP only (EV=empty vector), ad-ILK WT (ILK WT ) and ad-ILK R211A (ILK R211A ). Asterisks indicate high dispersion of R–R intervals, quantitated as chaos entropy coefficients: EV=−0.09; ILK=0.396; R211A=1.96. P(Mann–Whitney, for ILK and R211A versus EV) <0.05. ( d ) Reduction in impedance signal amplitude denoted by cell index (CI) of iPSC-CMs with the addition of DOX; treatments same as in c , * P <0.05, by Student’s t -test. ( e ) Changes in beat rate of iPSC-CMs with DOX; treatments same as in c . * P <0.05 by Student’s t -test. Error bars represent mean±s.e.m. Full size image DOX administration in vivo reduced expression levels of ILK, SERCA-2a and pPLN ( Supplementary Fig. 5a ). This effect was attenuated in ILK R211A compared with littermate control mice, as was the rate of apoptosis ( Supplementary Fig. 5b ). Importantly, improved sarcomeric architecture specific to the ILK R211A hearts was also seen 5 days post-DOX exposure ( Supplementary Fig. 6a,b ). DOX exposure has been reported to increase heart rate variability (HRV) and decrease contractility amplitude in murine iPSC-derived cardiac myocytes based upon real-time impedance monitoring [52] . The firing rates and contractility profiles of iPSC-CMs transduced with either ILK WT or ILK R211A constructs were determined at 24 h following DOX exposure by measurements of electrical impedance using the RTCA Cardio System. DOX exposure increased the dispersion of R–R intervals calculated as chaos entropy coefficients, an effect that was significantly attenuated following ILK transductions ( Fig. 4c ). This result is in agreement with the reduction in provokable ventricular arrhythmias observed following SERCA-2a gene therapy in a swine infarction model attributable to stabilization of SR calcium loading [53] . Transduction of ILK R211A protected against the DOX-induced amplitude reduction of the impedance signal in iPSC-CMs compared with that in ILK WT -transduced cells ( Fig. 4d ), which is consistent with the comparatively greater increase in releasable SR calcium content noted in iPSC-CMs transduced with ILK R211A ( Supplementary Fig. 4 ). ILK WT and ILK R211A caused an increase in cardiomyocyte firing rates pre- and post-DOX exposure compared with vector-only transduced control cells ( Fig. 4e ). The depressive effects of DOX on cardiac function in vivo were compared in ILK R211A and ILK WT transgenic mice using echocardiography. In line with the results observed following DOX exposure in vitro , preservation of cardiac function based on LV-shortening fraction was better in the ILK R211A genotype compared with that of the ILK WT transgenic mice determined 5 days following 20 mg per kg/ip DOX administration ( Supplementary Fig. 7 ). Together, this analysis indicates that the ILK R211A mutation and ILK WT resulted in relative preservation of heart rate and rhythm of human iPSC-CMs in response to DOX, whereas preservation of contractility was enhanced by overexpression of the ILK R211A mutation in vitro and in vivo . Our data suggest a model in which ILK serves as a mechanoreceptor for the transduction of increased contractility and for modulation of cardiomyocyte relaxation (lusitropy) through a newly identified interaction with SERCA-2a and PLN. Thus, ILK–SERCA–2a-PLN interaction provides a mechanism through which mechanoreception is dynamically linked to calcium regulation at the sarcomeric level. Our findings in myocardium representing advanced DCM revealed an increase in mRNA levels of ILK and ATP2A without proportional increases in their corresponding protein expression levels. These results imply post-transcriptional regulation of ILK and SERCA-2a protein that is specific to DCM. Z-disk colocalization of ILK with SERCA-2a/PLN was demonstrated in control human myocardium, which we hypothesize represents an adhesion-dependent mechanoreceptor complex that may also represent a disease target for degradation in DCM. Conversely, in normal human cardiomyocytes that are not subject to adverse processes inherent to DCM, the overexpression of ILK resulted in corresponding increases in ILK and SERCA-2a protein levels. The capacity of ILK to co-IP with SERCA-2a and PLN in transgenic myocardium ( Supplementary Figs 1 and 3 ) and the direct correlation between the protein but not mRNA expression levels of ILK and SERCA-2a following modulated ILK expression in iPSC-CMs ( Supplementary Fig. 2 ) suggest a model in which ILK and SERCA-2a comprise a protein-binding-dependent module. SERCA-2a is a widely validated molecular target in experimental and clinical heart failure that may be subject to downregulation [7] , [20] , [54] or adverse post-translational modifications including nitration [55] . Overexpression of ILK, using for example gene therapy, would nevertheless be expected to increase SERCA-2a/PLN function and thereby improve cardiac function in DCM through a protein-binding-dependent mechanism, irrespective of the primary inciting process. The role of CaMKII activation in heart failure has been interpreted as adverse [56] or beneficial and compensatory [20] , [57] , and the net phenotypic outcome may be dependent upon concomitant activation of interacting signalling pathways. For example, CaMKII signalling may be opposed by activation of calcineurin (Cn)/nuclear factor of activated transcription (NFAT) signalling in a time- and context-dependent manner such that Cn/NFAT signalling and activation (dephosphorylation) of GSK-3β may dominate that of CaMKII only following the transition from adaptive to adverse hypertrophic remodelling [58] . Although the effects of ILK on Cn/NFAT activation were not investigated in our studies, Cn/NFAT activation appears to be a feature of the ischaemic but not the dilated form of human cardiomyopathy [59] . One caveat is that SERCA-2a/PLN-dependent changes in the spontaneous cardiomyocyte beat rate in response to modulated ILK expression demonstrated in vitro cannot be directly translated to predicted chronotropic effects in vivo , which are instead governed by intrinsic pacemaker activation located electrophysiologically proximal to the level of ventricular myocytes. Our findings indicate that SERCA-2a function is enhanced through a dual mechanism that is stimulated by ILK overexpression, featuring increases in the protein level of SERCA-2a and Thr17 phosphorylation of PLN, both of which act to augment SR calcium ion pump flux. Multidomain adaptor proteins such as ILK typically regulate cellular signal transduction pathways through leveraged interactions with other adaptor proteins and protein kinases [60] . We have demonstrated that both endogenous ILK and exogenous ILK WT and ILK R211A establish protein–protein interactions with SERCA-2a, suggesting that SERCA-2a elevation resulting from ILK transduction is protein-binding-dependent. We have also shown that the anti-apoptotic effects of ILK (WT and R211A) against DOX-induced cardiotoxicity were not abrogated by the PI3K inhibitor LY294002 or by ILK kinase inhibition. Taken together, our results support a mechanotransduction pathway actuated by ILK scaffolding function that minimally involves CamKII, SERCA-2a, PLN and GSK-3β ( Fig. 5 ). A scaffolding mechanism is consistent with the mode of action of ILK described in the nucleation of multiprotein complexes at the site of focal adhesion formation in non-cardiac cell types [32] , [35] , [61] . 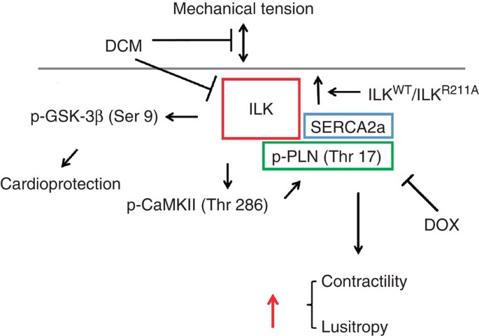Figure 5: ILKWTand ILKR211Aactivate SERCA-2a/PLN regulatome function. Model showing signalling pathway regulated by ILK, which is activated in response to mechanical tension developed across contiguous cardiomyocytes. ILK nucleates protein complexes leading to phosphorylation of components in this pathway (CaMKII, PLN and GSK-3β) that, in turn, regulate the functions of SERCA-2a and GSK-3β. SERCA-2a/PLN determines cardiac contractility and relaxation; phosphorylation of GSK-3β mediates cardioprotection against stress. Force transduction and the activation state of this pathway are decreased in DCM, and can be rescued by ILK (WT and R211A) overexpression. Figure 5: ILK WT and ILK R211A activate SERCA-2a/PLN regulatome function. Model showing signalling pathway regulated by ILK, which is activated in response to mechanical tension developed across contiguous cardiomyocytes. ILK nucleates protein complexes leading to phosphorylation of components in this pathway (CaMKII, PLN and GSK-3β) that, in turn, regulate the functions of SERCA-2a and GSK-3β. SERCA-2a/PLN determines cardiac contractility and relaxation; phosphorylation of GSK-3β mediates cardioprotection against stress. Force transduction and the activation state of this pathway are decreased in DCM, and can be rescued by ILK (WT and R211A) overexpression. Full size image Both wild-type and ILK R211A genes offer potential advantages compared with SERCA-2a gene therapy [5] , based on their capacity to enhance SERCA-2a function through phosphorylation of PLN, and also to promote cardioprotection through collateral activation of prosurvival pathways [62] , [63] . The ILK R211A transgenic mouse is resistant to angiotensin II-induced adverse cardiac hypertrophy [15] and, moreover, is not oncogenic when overexpressed, suggesting that the ILK R211A mutant is a potentially superior gene therapy candidate. Our data indicate that the ILK R211A mutation imparts gain-of-function in terms of cardiac contractility relative to ILK WT , including increased releasable SR calcium content in cardiac myocytes expressing the ILK R211A mutant. The apparent gain-of-function seen with ILK R211A may be explainable on the basis of higher expression levels of ILK and SERCA-2a compared with that resulting from ILK WT overexpression, which were consistently observed following both adenoviral transduction using the same multiplicity of infection dosage in vitro and in transgenic mice in vivo . We previously reported that ILK R211A expression results in a heat-shock protein chaperone response [64] . Notably, Hsp90 has been also shown to stabilize ILK-containing protein complexes in non-cardiac cells through inhibition of proteolytic degradation [61] , [65] . A clinically relevant issue to be addressed in future studies is to determine the corresponding cardiac phenotypes resulting from gene therapy implementations employing ILK WT versus ILK R211A constructs. In light of the emerging renaissance of gene therapy in the treatment of heart failure [5] , [66] , adeno-associated viral delivery of ILK R211A by coronary artery injection can be envisioned for patients with advanced DCM on ventricular assist devices awaiting transplantation. More broadly, our findings advance the theme that engineered mutations in cytoprotective protein kinases can be exploited to help separate their cytoprotective and potentially oncogenic properties. Generation of transgenic mice and adenoviral constructs The methods for generation of transgenic animals conveying cardiac-specific overexpression of ILK WT and mutant (ILK R211A ) versions of the human ILK gene on a C57BL/6 background have been previously described [15] . Male transgenic mice and littermate controls 2–3 months of age were used for the experiments. Genotypes were confirmed in all mice using KAPA Mouse Genotyping Kit (KAPA BIOSYSTEMS, KK7302). DOX (doxorubicin hydrochloride, catalogue number: D1515, Sigma-Aldrich) was administered to 10-week-old Tg R211A C57BL/6J mice and their littermate controls by a single intraperitoneal injection at a dose of 20 mg kg −1 . Research ethics board approval The Animal Care Committee at the Hospital for Sick Children, which operates in accordance with the Terms of Reference following the Canadian Council on Animal Care Guidelines and federal and provincial regulations/legislations, gave approval to this study. Human myocardial samples were acquired with approval of the Research Ethics Board protocols under the auspices of the Heart Centre Biobank Registry (no. 1000011232; no. 1000011017; no. 1000032470). Each subject gave signed informed consent to tissue analysis. Immunohistochemical analysis Six-micrometre-thick cryosections were cut across the muscle, fixed in 4% paraformaldehyde for 20 min at room temperature, rinsed with phosphate-buffered saline (PBS) and then permeabilized with 0.1% Triton-X 100 in PBS for 10 min. After permeabilization the slides were blocked with 5% milk in PBS for 30 min and subjected to immunostaining with appropriate primary antibody for 2 h. The following primary antibodies were used: ILK (catalogue number: 3856, Cell Signaling Technology, 1:200 dilution), SERCA-2a (2A7-A1; catalogue number: ab2861, Abcam, 1:100 dilution), α-actinin (sarcomeric; catalogue number: A7811, Sigma-Aldrich, 1:800 dilution), total PLN (2D12; catalogue number: MA3-922, Thermo Scientific, 1:100 dilution) and cardiac Troponin T (13-11; catalogue number: MA5-12960, Thermo Scientific, 1:100 dilution). After incubation with the primary antibody the cryosections were washed with PBS and then incubated for 1 h with fluorescent-conjugated secondary antibody (Jackson ImmunoResearch Laboratories). Nuclei were stained with 4′,6-diamino-2-phenylindole. The mounted sections were observed using a Spinning Disk Confocal Microscope and then analysed using the Volocity software. Apoptosis assay The presence of apoptosis-related DNA strand breaks in Hu iPS-CMs was evaluated using the terminal deoxynucleotidyl transferase end labelled nucleotide (TUNEL) assay using the In situ Cell Death Detection kit, POD (Roche Molecular Biochemicals, Mannheim, Germany) according to the manufacturer’s instructions. In short, cells on coverslips were maintained in culture and then fixed with 4% paraformaldehyde for 20 min at room temperature. Following rinsing with PBS, cells were permeabilized with 0.1% Triton-X 100 (Sigma) for 10 min and then supplemented with 3% H 2 O 2 to quench endogenous peroxidase activity. Thereafter, cells were incubated with TUNEL reaction mixture. Next, cells were rinsed in PBS and incubated with Converter-POD (anti-fluorescein antibody conjugated with horseradish peroxidase). Peroxidase activity was then visualized by precipitation of DAB (DAB Substrate, Roche). Cells containing fragmented nuclear chromatin exhibited a brown nuclear stain. As negative controls, sections were processed without terminal deoxynucleotidyltransferase (TdT) buffer. Apoptotic cells were examined with a Leica DMR microscope. The number of TUNEL-positive cells was counted in at least 10 random fields per treatment. Western blotting Total and phospho-specifc protein expression was measured in lysates derived from human iPSC-derived cardiomyocytes in culture and from transgenic and control mouse or human ventricular tissues. Cells/tissue extracts were prepared by lysing the cells for 20 min on ice in RIPA lysis buffer (150 mM NaCl, 1% Nonidet P40, 05% deoxycholate, 0.1% SDS, 50 mM Tris, pH 8.0 and 1 mM phenylmethylsulphonyl fluoride). The expression levels of the proteins were assessed using the following antibodies: ILK (catalogue number: 3,856, Cell Signaling Technology, 1:2,000 dilution), GAPDH (catalogue number: G8795, Sigma-Aldrich, 1:5,000 dilution), total GSK-3β (catalogue number: 9315, Cell Signaling Technology, 1:1,000 dilution), phospho-GSK-3β (Ser9; catalogue number: 9323, Cell Signaling Technology, 1:1,000 dilution), SERCA-2a (2A7-A1; catalogue number: ab2861, Abcam, 1:1,000 dilution), phospho-CaMKIIα (Thr 286; catalogue number: 12,886-R, Santa Cruz Biotechnology Inc., 1:1,000 dilution), total CamMKII (G-1; catalogue number: sc-5306, Santa Cruz Inc., 1:800 dilution), phospho-PLN (Thr 17)-R (catalogue number: sc-17,024-R, Santa Cruz Biotechnology Inc., 1:800 dilution) and total PLN (2D12; catalogue number: MA3-922, Thermo Scientific, 1:1,000 dilution). After incubation with the primary antibody, the blots were washed and incubated for 1 h with the appropriate horseradish peroxidase-conjugated secondary antibody (Jackson ImmunoResearch Laboratories, 1:5,000 dilution). Proteins were visualized by chemiluminescence using either SuperSignal West Pico substrate (Pierce) or SuperSignal West Dura Extended Duration Substrate (Pierce). Administration and doses of chemicals Thapsigargin (Sigma) was used at 1 μM. CaMKII inhibitor KN-93 (catalogue number: 2,02,199, Santa Cruz Biotechnology Inc.) and inactive analogue KN-92 (catalogue number: 3,11,369, Santa Cruz Biotechnology Inc.) were used at 1 μM. PI3K inhibitor LY294002 (catalogue number: 9,901, Cell Signaling Technology) was used at 30 μM. ILK inhibitor QLT0267 (obtained as a gift from Dr Shoukat Dedhar) was used at 20 μM. Real-time quantitative PCR RNA was isolated using the Direct-zol RNA MiniPrep kit (Zymo Research). First-strand cDNA synthesis was synthesized from 1 μg of RNA using qScriptcDNA Supermix (Quanta BioSciences) and SuperScript VILOcDNA Synthesis Kit (Life Technologies). SYBR green and Taqman methods were used with the Bio-Rad CFX96 Touch Real-Time PCR Detection System. SYBR green and Taqman qPCR data were normalized to the housekeeping genes, GAPDH and TBP , respectively. Primers and probes are listed in Supplementary Table 1 . RNA interference, transfection and transduction siRNA against ILK (siILK) and negative control siRNA were purchased from Cell Signaling Technologies. Cells were transfected with siRNAs (130 μM final concentration) using the X-tremeGENE siRNA transfection reagent (Roche Diagnostics, Laval, QC, Canada) according to the manufacturer’s instructions. To increase transduction efficiency the cells were transfected again after 24 h with the same concentration of siRNA. The cells were analysed at 48 h post transfection. Cardiomyocytes derived from human iPSC-CMs Cryopreserved IPSC-CMs (catalogue no. CMC-100-110-001, Cellular Dynamics International) were thawed and cultured on plastic dishes (coated with 0.1% gelatin) in plating medium (catalogue no. CMM-100-110-001). After 2 days the cultured medium was replaced with maintenance medium (catalogue no. CMM-100-210-001) for 5 more days before ILK adenoviral infection as described [15] . Cardiomyocytes were confirmed to contract synchronously at greater than 80% confluency. Mass spectrometry The mass spectrometric experiments were performed using an on-line liquid chromatography-tandem mass spectrometry set-up using an Agilent 1100 Capillary LC system (Palo Alto, CA, USA) fitted to a LTQ ion trap mass spectrometer (Thermo Electron, San Jose, CA, USA). A C18 pre-column (100 μm i.d. × 5.0 cm length) and a μLC analytical column (75 μm × 10 cm) that also served as a μESI emitter were used for the separation of the digested proteins. The mass spectrometer was operated in data-dependent mode automatically cycling through acquisition of a full-scan mass spectrum and three MS/MS spectra recorded sequentially on the three most abundant ions present in the initial MS scan. A dynamic exclusion list time of 1.5 min was used. For the reverse phase chromatography, an 80-min gradient elution from water to acetonitrile, each containing 0.1% FA and 0.02% TFA, was performed at a flow of 200 nl min −1 . All MS/MS spectra were searched against the NCBInr protein database using MASCOT Server (v2.2; Matrix Science). The search results were analysed using the Scaffold software (Proteome software). The mass spectrometry proteomics data have been deposited to the ProteomeXchange Consortium via the PRIDE partner repository with the data set identifier PXD001053. Measurements of calcium transients in iPSC-CMs Cardiomyocytes were loaded with Rhodamine-3, a red-shifted calcium dye [67] . The cells were stained according to the protocol provided by the manufacturer (Invitrogen) and imaged using a Zeiss Axiovert 100 M Confocal Microscope. A line scan image of each cell was taken and converted to an intensity versus time graph. To minimize potential effects of variability in time-related flourescence decay, the sequencing of calcium imaging corresponding to each adenoviral construct was performed using enforced randomization such that each construct was imaged as the first through fourth target cell 24 h post transfection. Three consecutive peaks from each graph were chosen for further analysis examining parameters including amplitude, time to peak, decay time, rate of transients and time constant tau ( τ ), determined using Origin 8.0 (Origin Labs). xCelligence Cardiomyocytes derived from IPSC-CMs were plated into 96-well plates designed for the xCelligence RTCA Cardio instrument ( http://www.roche-applied-science.com/sis/xcelligence/ ) at a density of 10,000 cells per well. The cells were grown for 4 days until regular, synchronized beating was observed across all wells. Adenoviruses encoding for empty vector (control), ILK and ILK-R211A were transfected into the myocytes as described above. Thapsigargin (1 μ M ; Sigma) or DOX (1 μM) were added to the wells as indicated maintaining the plate and cells at 37 °C to avoid any effect of temperature changes or cellular removal from the incubator on the myocytes. Heart rate variability The beat-to-beat variation was quantified by measuring the time between successive peaks on the impedance tracings obtained from the xCELLigence RTCA cardio instrument before (1 h) and after (24 h) treatment with doxorubicin. The beat-to-beat time periods were subjected to a Poincare analysis to quantify HRV. The encompassing oval method of Poincare plot reduction [68] was used to generate a single metric of irregularity referred to as chaos entropy coefficient. Each condition was performed in triplicate and the results were compared using a Mann–Whitney test to generate a P value. Mouse echocardiography Echocardiographic studies were performed under conditions of 1–2% isoflurane anaesthesia with spontaneous ventilation. The Vevo 770 high-resolution Micro-Ultrasound system with RMV 707B transducer (Visualsonics Inc., Toronto) were used to acquire two-dimensional (2D) images and M-mode measurements using the parasternal long axis view; pulse wave Doppler and tissue Doppler imaging relied on a modified apical four-chamber view. Image acquisition and analysis were performed by readers blinded as to treatment group, and informally randomized as to genotype. Indices were calculated on data averaged from a minimum of three consecutive cardiac cycles wherever possible. The myocardial performance index [69] or the Tei index of the LV was calculated using Doppler flow intervals as follows: Tei index=isovolumic contraction time+isovolumic relaxation time)/LV ejection time. All measurements were calculated with the VEVO Analysis software (version 2.2.3). Statistical analyses Data are provided as mean±s.e.m. Statistical analysis was carried out by using two-tailed Student’s t -test or the Mann–Whitney to test for differences in the distribution of HRV data. Significance was accepted at P <0.05. How to cite this article: Traister, A. et al. Integrin-linked kinase mediates force transduction in cardiomyocytes by modulating SERCA2a/PLN function. Nat. Commun. 5:4533 doi: 10.1038/ncomms5533 (2014). Accession codes: Mass spec data have been deposited in ProteomeXchange under accession code PXD001053.